Regulation of MKL1 via actin cytoskeleton dynamics drives adipocyte differentiation Cellular differentiation is regulated through activation and repression of defined transcription factors. A hallmark of differentiation is a pronounced change in cell shape, which is determined by dynamics of the actin cytoskeleton. Here we show that regulation of the transcriptional coactivator MKL1 (megakaryoblastic leukemia 1) by actin cytoskeleton dynamics drives adipocyte differentiation mediated by peroxisome proliferator–activated receptor γ (PPARγ), a master transcriptional regulator of adipogenesis. Induction of adipocyte differentiation results in disruption of actin stress fibres through downregulation of RhoA-ROCK signalling. The consequent rapid increase in monomeric G-actin leads to the interaction of G-actin with MKL1, which prevents nuclear translocation of MKL1 and allows expression of PPARγ followed by adipogenic differentiation. Moreover, we found that MKL1 and PPARγ act in a mutually antagonistic manner in the adipocytic differentiation programme. Our findings thus provide new mechanistic insight into the relation between the dynamics of cell shape and transcriptional regulation during cellular differentiation. Activation and repression of defined transcription factors are essential for the commitment of progenitors to a specific differentiation lineage, setting the stage for a gene expression pattern characteristic of each mature cell type [1] , [2] , [3] . Adipocyte differentiation is regulated by multiple transcription factors, with PPARγ and members of the CCAAT/enhancer-binding protein (C/EBP) family having central roles. Cooperative interactions among these transcription factors drive the expression of downstream target genes that are necessary for the generation and maintenance of adipocyte characteristics such as lipid accumulation and insulin sensitivity [4] . The key role of PPARγ in the commitment of mesenchymal precursors to the adipocytic differentiation programme is evident from the observation that forced expression of this protein stimulates adipogenesis in nonadipogenic fibroblastic cell lines, such as NIH 3T3 and 3T3-C2 (refs 5 , 6 ). PPARγ is thus thought to function as an adipocyte-specific master switch in acquisition of the adipocytic phenotype [7] . The adipocytic differentiation of fibroblastic preadipocytes is accompanied by the adoption of a rounded morphology that is characteristic of mature adipocytes and allows for maximal lipid storage [8] . Cell morphology is determined primarily by the actin cytoskeleton [9] . Adipocyte differentiation is thus associated with a shift in the structures formed by filamentous (F) actin from stress fibres to cortical fibres [10] , [11] . The relation between such reorganization of the actin cytoskeleton and the PPARγ-mediated adipocytic differentiation programme has remained unclear, however. We have previously established a preadipocyte cell line derived from mouse dedifferentiated fat (DFAT) cells and which possesses a higher potential to differentiate into adipocytes compared with the mouse preadipocyte cell line 3T3-L1 (ref. 12 ). Unlike 3T3-L1 cells, these DFAT cells do not undergo spontaneous adipogenesis, with the adipocytic differentiation of DFAT cells thus being more tightly controlled than that of 3T3-L1 cells [12] , [13] . Here, we examine the roles of actin cytoskeleton remodelling in adipocytic differentiation by using DFAT cells. We show that the rapid disruption of actin stress fibres through downregulation of RhoA-ROCK signalling and the consequent increase in monomeric G-actin levels are observed before adipocyte differentiation. We also found that interaction of monomeric G-actin with the transcriptional coactivator MKL1 is the key event for initiating PPARγ expression. Moreover, MKL1 and PPARγ were shown to act in a mutually antagonistic manner in the adipocytic differentiation programme. Our findings provide a new insight into the regulatory mechanism of adipocyte differentiation. Adipogenesis requires disruption of actin stress fibres We first examined the changes in the actin cytoskeleton and PPARγ expression during adipogenesis with the use of an established DFAT cell line. Before induction of adipogenesis, DFAT cells manifest a fibroblastic morphology with well-developed actin stress fibres ( Fig. 1a ). At 24 h after the induction of adipocytic differentiation with the combination of 3-isobutyl-1-methylxanthine (IBMX), dexamethasone and insulin, the cells exhibit a well-spread morphology associated with the disruption of most stress fibres ( Fig. 1a,c ; Supplementary Movie 1 ). The upregulation of PPARγ expression at both mRNA and protein levels is evident at 48 h ( Fig. 1a,b ), at which time the cell morphology has become stellate and the cortical actin structures characteristic of adipocytes are evident ( Fig. 1a ). The expression of perilipin (a marker of terminal adipocyte differentiation) and the accumulation of lipid droplets are observed from 60 h, at which time the cell morphology has become more rounded ( Fig. 1a ). Together, these results thus suggested that disruption of actin stress fibres precedes the induction of PPARγ expression during adipocyte differentiation. 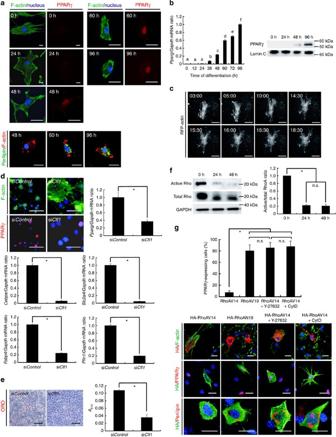Figure 1: Disruption of actin stress fibres is required for adipocyte differentiation. (a) Fluorescence microscopy of the actin cytoskeleton (stained with phalloidin) as well as of PPARγ or perilipin expression during adipogenesis in DFAT cells. Nuclei were stained with Hoechst 33342 (blue fluorescence). Scale bars, 20 μm. (b) Relative abundance ofPpargmRNA during adipocytic differentiation in DFAT cells (left panel). (a–f)P<0.05, Tukey’s honest significant difference test. A nuclear fraction prepared from the cells was also subjected to immunoblot analysis of PPARγ and lamin C (loading control) (right panel). (c) Time-lapse imaging of DFAT cells expressing red fluorescent protein (RFP)–tagged actin at the indicated times (hours:minutes). Scale bars, 50 μm. (d) 3T3-L1 preadipocytes transfected with cofilin1 (siCfl1-a) or control (siControl) siRNAs were exposed to inducers of differentiation for 96 h. They were then subjected to fluorescence microscopic analysis of the actin cytoskeleton and PPARγ expression. Nuclei were stained with Hoechst 33342. Scale bars, 50 μm. Relative abundance ofPparg,Cebpa,Fabp4,Slc2a4andPlin1mRNAs. *P<0.05, Student’st-test. (e) Oil red O (ORO) staining of cells treated as ind. Bars, 100 μm. The absorbance at 510 nm (A510) of dye extracted from the stained cells was also determined. *P<0.05, Student’st-test. (f) Immunoblot analysis of active and total forms of Rho proteins during adipocyte differentiation in DFAT cells (left panels). GAPDH was examined as a loading control. Quantification of the immunoblotting data was performed using densitometry. Data were normalized to the amount of total Rho (right panel). *P<0.05, Student’st-test. n.s., not significant. (g) Fluorescence microscopy of the actin cytoskeleton as well as of PPARγ or perilipin expression in DFAT cells expressing HA-tagged RhoAV14 or RhoAN19 and exposed for 96 h to inducers of differentiation in the absence or presence of Y-27632 (30 μM) or CytD (0.2 μM). Nuclei were stained with Hoechst 33342. Scale bars, 20 μm. At least 50 HA-positive cells were scored for determination of the percentage of those expressing PPARγ. *P<0.05, Student’st-test. All quantitative data are means±s.d. (n=3 experiments fibres). Figure 1: Disruption of actin stress fibres is required for adipocyte differentiation. ( a ) Fluorescence microscopy of the actin cytoskeleton (stained with phalloidin) as well as of PPARγ or perilipin expression during adipogenesis in DFAT cells. Nuclei were stained with Hoechst 33342 (blue fluorescence). Scale bars, 20 μm. ( b ) Relative abundance of Pparg mRNA during adipocytic differentiation in DFAT cells (left panel). ( a – f ) P <0.05, Tukey’s honest significant difference test. A nuclear fraction prepared from the cells was also subjected to immunoblot analysis of PPARγ and lamin C (loading control) (right panel). ( c ) Time-lapse imaging of DFAT cells expressing red fluorescent protein (RFP)–tagged actin at the indicated times (hours:minutes). Scale bars, 50 μm. ( d ) 3T3-L1 preadipocytes transfected with cofilin1 (si Cfl1 -a) or control (si Control ) siRNAs were exposed to inducers of differentiation for 96 h. They were then subjected to fluorescence microscopic analysis of the actin cytoskeleton and PPARγ expression. Nuclei were stained with Hoechst 33342. Scale bars, 50 μm. Relative abundance of Pparg , Cebpa , Fabp4 , Slc2a4 and Plin1 mRNAs. * P <0.05, Student’s t -test. ( e ) Oil red O (ORO) staining of cells treated as in d . Bars, 100 μm. The absorbance at 510 nm ( A 510 ) of dye extracted from the stained cells was also determined. * P <0.05, Student’s t -test. ( f ) Immunoblot analysis of active and total forms of Rho proteins during adipocyte differentiation in DFAT cells (left panels). GAPDH was examined as a loading control. Quantification of the immunoblotting data was performed using densitometry. Data were normalized to the amount of total Rho (right panel). * P <0.05, Student’s t -test. n.s., not significant. ( g ) Fluorescence microscopy of the actin cytoskeleton as well as of PPARγ or perilipin expression in DFAT cells expressing HA-tagged RhoAV14 or RhoAN19 and exposed for 96 h to inducers of differentiation in the absence or presence of Y-27632 (30 μM) or CytD (0.2 μM). Nuclei were stained with Hoechst 33342. Scale bars, 20 μm. At least 50 HA-positive cells were scored for determination of the percentage of those expressing PPARγ. * P <0.05, Student’s t -test. All quantitative data are means±s.d. ( n =3 experiments fibres). Full size image Previous studies have shown that actin cytoskeleton dynamics associated with cell rounding in response to mechanical or physical stimuli (such as matrix stiffness and cytoskeletal tension) result in adipogenic differentiation of 3T3-F442A preadipocytes or mesenchymal stem cells by a mechanism that involves RhoA-ROCK (Rho-kinase) signalling [14] , [15] , [16] , [17] , [18] , which regulates the formation of actin stress fibres and focal adhesions [19] , [20] . On the other hand, ectopic expression of PPARγ in mesenchymal stem cells or NIH 3T3 fibroblasts has been found to induce not only expression of adipose-specific genes but also morphological differentiation, including the accumulation of triglyceride droplets [5] , [21] , [22] , [23] , [24] . It has remained unknown, however, whether the pathways underlying the induction of adipogenesis either by PPARγ or by changes in cell shape operate independently of each other or in an interdependent manner. To address this question, we tested the effects both of RNA interference (RNAi)-mediated depletion of cofilin1, a protein that promotes the disassembly of actin filaments [25] , and of phalloidin (a cytoskeletal fixative) on PPARγ expression during adipocyte differentiation. Either knockdown of cofilin1 with specific small interfering RNAs (siRNAs) or treatment with phalloidin blocked the disruption of actin stress fibres as well as markedly inhibited both the upregulation of PPARγ and PPARγ target gene expression and the accumulation of lipid droplets elicited by inducers of adipocyte differentiation in DFAT cells and 3T3-L1 preadipocytes ( Fig. 1d,e ; Supplementary Fig. 1 ). These data thus indicated that the disruption of actin stress fibres is required for the induction of PPARγ expression during adipocyte differentiation. RhoA-ROCK signalling regulates adipogenesis We next investigated whether RhoA-ROCK signalling plays a role in adipogenic differentiation dependent on the disruption of actin stress fibres in DFAT cells. The GTP-bound (active) form of Rho proteins was detected at a high level before adipogenic induction and was markedly reduced in abundance within 24 h after exposure of the cells to inducers of adipocyte differentiation ( Fig. 1f ). We transiently transfected DFAT cells with plasmids encoding hemagglutinin epitope (HA)–tagged dominant active (RhoAV14) or dominant negative (RhoAN19) mutants of RhoA and then exposed the cells to inducers of adipocytic differentiation for 96 h. Expression of RhoAV14 inhibited both remodelling of the actin cytoskeleton as well as the induction of PPARγ and perilipin expression, and these inhibitory effects were prevented by treatment with the ROCK inhibitor Y-27632 ( Fig. 1g ). We also determined whether the effects of ROCK inhibition in RhoAV14-expressing cells were mimicked by the actin-depolymerizing agent cytochalasin D (CytD). The addition of CytD indeed restored remodelling of the actin cytoskeleton as well as the expression of PPARγ and perilipin in RhoAV14-expressing cells to levels similar to those apparent in RhoAV14-expressing cells treated with Y-27632 or in cells expressing RhoAN19 ( Fig. 1g ). These results thus indicated that RhoA-ROCK signalling regulates adipocyte differentiation through control of remodelling of the actin cytoskeleton. G-actin induces adipogenesis by controling MKL1 localization Recent studies have identified mechanisms by which actin dynamics directly affect gene transcription [26] . Monomeric G-actin binds to the transcriptional coactivator MKL1 (also known as MAL or MRTF-A) and prevents it from translocating to the nucleus and activating transcription [27] , [28] . Furthermore, in multipotent mesenchymal stem cells, Med23 functions as a molecular switch between ELK1 and MKL1 that controls differentiation into adipocytes or smooth muscle cells [29] , suggesting links between MKL1 and adipogenesis. To explore whether the control of MKL1 translocation by cellular G-actin contributes to the regulation of PPARγ expression and adipocyte differentiation, we established DFAT cells expressing mCherry fused to MKL1 (mCherry-MKL1; Supplementary Fig. 2a ) and investigated G-actin levels and mCherry-MKL1 localization before and after the induction of adipocyte differentiation. F-actin was rapidly depolymerized to monomeric G-actin after the induction of adipocyte differentiation, with the increase in cellular G-actin concentration ( Fig. 2a ). mCherry-MKL1 was detected exclusively in the nucleus before adipogenic induction but was predominantly pancellular and/or cytoplasmic after the induction of adipogenesis ( Fig. 2a ). PPARγ expression was detected in cells having the cytoplasmic localization of mCherry-MKL1 ( Supplementary Fig. 2b ). 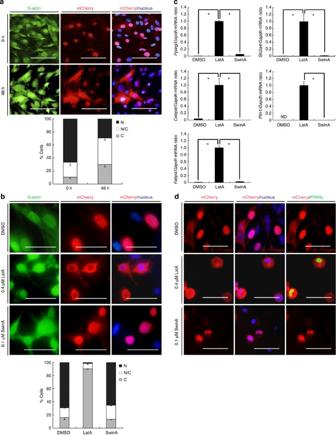Figure 2: The increase of G-actin accumulation resulting from disruption of actin stress fibres is involved in the cytoplasmic sequestration of MKL1 and adipocyte differentiation in DFAT cells. (a) Immunofluorescence analysis of mCherry and G-actin (stained with DNase I) in cells stably expressing mCherry-MKL1 at 0 or 48 h after the induction of adipogenesis(upper panels). Nuclei were stained with Hoechst 33342. Scale bars, 100 μm. At least 300 cells per coverslip were scored for determination of the percentage of the subcellular localization of MKL1 (lower panel). N, nuclear; N/C, comparable intensity in nucleus and cytoplasm; C, cytoplasmic. (b) Immunofluorescence analysis of mCherry and G-actin in mCherry-MKL1-expressing cells exposed to Lat A (0.4 μM), Swin A (0.1 μM) or dimethyl sulfoxide (DMSO, control) for 6 h in growth medium without an adipogenic cocktail (upper panels). Nuclei were stained with Hoechst 33342. Scale bars, 50 μm. Quantitation of immunofluorescence microscopy; localization of the indicated mCherry-MKL1 was scored in 300 cells as in panela(lower panel). (c) Relative abundance ofPparg,Cebpa,Fabp4,Slc2a4, andPlin1mRNAs in cells treated as inb. ND, not detected. (d) Cells treated as inbwere cultured for an additional 18 h (total of 24 h) and then subjected to immunofluorescence analysis of mCherry and PPARγ expression. Nuclei were stained with Hoechst 33342. Scale bars, 50 μm. All quantitative data are means±s.d. (n=3 experiments). *P<0.05, Student’st-test. Figure 2: The increase of G-actin accumulation resulting from disruption of actin stress fibres is involved in the cytoplasmic sequestration of MKL1 and adipocyte differentiation in DFAT cells. ( a ) Immunofluorescence analysis of mCherry and G-actin (stained with DNase I) in cells stably expressing mCherry-MKL1 at 0 or 48 h after the induction of adipogenesis(upper panels). Nuclei were stained with Hoechst 33342. Scale bars, 100 μm. At least 300 cells per coverslip were scored for determination of the percentage of the subcellular localization of MKL1 (lower panel). N, nuclear; N/C, comparable intensity in nucleus and cytoplasm; C, cytoplasmic. ( b ) Immunofluorescence analysis of mCherry and G-actin in mCherry-MKL1-expressing cells exposed to Lat A (0.4 μM), Swin A (0.1 μM) or dimethyl sulfoxide (DMSO, control) for 6 h in growth medium without an adipogenic cocktail (upper panels). Nuclei were stained with Hoechst 33342. Scale bars, 50 μm. Quantitation of immunofluorescence microscopy; localization of the indicated mCherry-MKL1 was scored in 300 cells as in panel a (lower panel). ( c ) Relative abundance of Pparg , Cebpa , Fabp4 , Slc2a4 , and Plin1 mRNAs in cells treated as in b . ND, not detected. ( d ) Cells treated as in b were cultured for an additional 18 h (total of 24 h) and then subjected to immunofluorescence analysis of mCherry and PPARγ expression. Nuclei were stained with Hoechst 33342. Scale bars, 50 μm. All quantitative data are means±s.d. ( n =3 experiments). * P <0.05, Student’s t -test. Full size image We next tested whether actin-depolymerizing agents latrunculin A (LatA), which increases monomeric G-actin [27] , [30] , or swinholide A (SwinA), which increases dimeric actin that does not interact with MKL1 (refs 27 , 30 , 31 ), might mimic the effects of inducers of adipogenesis on dynamics of the actin cytoskeleton and MKL1 localization in DFAT cells expressing mCherry-MKL1. Indeed, LatA or SwinA induced disruption of actin stress fibres and increased the cellular abundance of G-actin monomers or dimers, respectively ( Fig. 2b ; Supplementary Fig. 2c ). LatA treatment caused the cytoplasmic sequestration of mCherry-MKL1, whereas SwinA treatment resulted in the nuclear localization ( Fig. 2b ). Furthermore, LatA alone induced a significant increase in the expression of PPARγ and PPARγ target genes unlike SwinA ( Fig. 2c,d ). These results suggested that monomeric G-actin formation leads to adipocyte differentiation by blocking the nuclear import of MKL1, but not by other consequences of disruption of actin stress fibres. Similarly to LatA, treatment with Y-27632, elicited disruption of actin stress fibres and the cytoplasmic sequestration of MKL1, resulting in a marked increase in the expression of PPARγ and PPARγ-target genes as well as in the accumulation of lipid droplets in DFAT cells and 3T3-L1 preadipocytes ( Supplementary Fig. 3 ). Adipogenesis requires interaction between G-actin and MKL1 We also asked whether the interaction between G-actin and MKL1 and the consequent cytoplasmic sequestration of MKL1 contribute to adipocyte differentiation. To address this issue, we established DFAT cells and 3T3-L1 preadipocytes that express a FLAG epitope–tagged fusion protein of the oestrogen receptor (ER) and either MKL1 or a deletion mutant of MKL1 (MKL1-N100) that lacks the 100 NH 2 -terminal amino acids of the full-length protein and therefore does not contain the RPEL actin-binding domain [32] , [33] ( Supplementary Fig. 4a ). Exposure of these cells to the ER agonist 4-hydroxytamoxifen (TAM) induced the nuclear translocation of each fusion protein ( Fig. 3a ). The nuclear translocation of ER-MKL1 was accompanied by a marked decrease in the expression of PPARγ and PPARγ target genes as well as in the accumulation of lipid droplets in cells also exposed to inducers of adipocytic differentiation ( Fig. 3b–d ; Supplementary Fig. 4b–d ). Moreover, expression of ER-MKL1-N100, which fails to bind G-actin and a substantial proportion of which was localized to the nucleus even in the absence of TAM ( Fig. 3b ; Supplementary Fig. 4b ), resulted in marked suppression of adipogenesis in the absence or presence of TAM compared with that apparent in cells expressing ER-MKL1 ( Fig. 3b–d ; Supplementary Fig. 4b–d ). We also tested if ER-MKL1-N100 reverts the effects elicited by treatment with LatA in DFAT cells and 3T3-L1 preadipocytes. The expression of ER-MKL1-N100, which was predominantly localized to the nucleus even after treatment with LatA and remarkably impaired the expression of PPARγ and PPARγ target genes compared with that of ER-MKL1 ( Fig. 3e,f ; Supplementary Fig. 4e,f ). These findings significantly strengthen our conclusion that the increase in the cytoplasmic abundance of G-actin triggers adipocyte differentiation via regulation of the subcellular localization of MKL1. 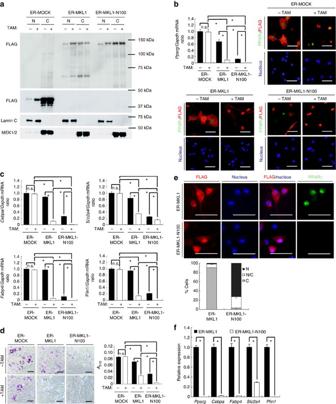Figure 3: Interaction between G-actin and MKL1 and the consequent cytoplasmic sequestration of MKL1 are required for adipocytic differentiation in DFAT cells. (a) Cells stably expressing 3 × FLAG-tagged ER (ER-MOCK, control), ER-MKL1 or ER-MKL1-N100 were exposed for 48 h to inducers of adipogenic differentiation in the absence or presence of TAM (1 μM), after which nuclear (N) and cytoplasmic (C) fractions were prepared from the cells and subjected to immunoblot analysis of FLAG, lamin C (nuclear marker) and MEK1/2 (cytoplasmic marker). (b) Cells treated as inawere analysed for the relative abundance ofPpargmRNA or subjected to immunofluorescence analysis of FLAG and PPARγ. Nuclei were stained with Hoechst 33342. Scale bars, 50 μm. (c) Relative abundance ofCebpa,Fabp4,Slc2a4andPlin1mRNAs in cells treated as ina. (d) Cells treated as inawere cultured for an additional 48 h (total of 96 h) and then stained with oil red O. Scale bars, 100 μm. TheA510of dye extracted from the stained cells was also determined. n.s., not significant. (e) Cells stably expressing ER-MKL1 or ER-MKL1-N100 were exposed for 24 h to Lat A (0.4 μM) in the presence of TAM (1 μM) and then subjected to immunofluorescence analysis of FLAG and PPARγ (upper panels). Nuclei were stained with Hoechst 33342. Scale bars, 50 μm. At least 300 cells per coverslip were scored for determination of the percentage of the subcellular localization of MKL1 (centre panel). N, nuclear; N/C, comparable intensity in nucleus and cytoplasm; C, cytoplasmic. (f) Relative abundance ofPparg,Cebpa,Fabp4,Slc2a4andPlin1mRNAs in cells treated as ine. All quantitative data are means±s.d. (n=3 experiments). *P<0.05, Student’st-test. Figure 3: Interaction between G-actin and MKL1 and the consequent cytoplasmic sequestration of MKL1 are required for adipocytic differentiation in DFAT cells. ( a ) Cells stably expressing 3 × FLAG-tagged ER (ER-MOCK, control), ER-MKL1 or ER-MKL1-N100 were exposed for 48 h to inducers of adipogenic differentiation in the absence or presence of TAM (1 μM), after which nuclear (N) and cytoplasmic (C) fractions were prepared from the cells and subjected to immunoblot analysis of FLAG, lamin C (nuclear marker) and MEK1/2 (cytoplasmic marker). ( b ) Cells treated as in a were analysed for the relative abundance of Pparg mRNA or subjected to immunofluorescence analysis of FLAG and PPARγ. Nuclei were stained with Hoechst 33342. Scale bars, 50 μm. ( c ) Relative abundance of Cebpa , Fabp4 , Slc2a4 and Plin1 mRNAs in cells treated as in a . ( d ) Cells treated as in a were cultured for an additional 48 h (total of 96 h) and then stained with oil red O. Scale bars, 100 μm. The A 510 of dye extracted from the stained cells was also determined. n.s., not significant. ( e ) Cells stably expressing ER-MKL1 or ER-MKL1-N100 were exposed for 24 h to Lat A (0.4 μM) in the presence of TAM (1 μM) and then subjected to immunofluorescence analysis of FLAG and PPARγ (upper panels). Nuclei were stained with Hoechst 33342. Scale bars, 50 μm. At least 300 cells per coverslip were scored for determination of the percentage of the subcellular localization of MKL1 (centre panel). N, nuclear; N/C, comparable intensity in nucleus and cytoplasm; C, cytoplasmic. ( f ) Relative abundance of Pparg , Cebpa , Fabp4 , Slc2a4 and Plin1 mRNAs in cells treated as in e . All quantitative data are means±s.d. ( n =3 experiments). * P <0.05, Student’s t -test. Full size image Loss of MKL1 drives adipocyte differentiation We further assessed whether RNAi-mediated depletion of MKL1 alone might induce PPARγ expression and adipocyte differentiation in the absence of an adipogenic cocktail. In both DFAT cells and 3T3-L1 preadipocytes, knockdown of Mkl1 expression ( Supplementary Fig. 5a ) resulted in a marked increase both in the expression of PPARγ and PPARγ target genes as well as in the extent of lipid droplet accumulation ( Fig. 4a ; Supplementary Fig. 5b,c ). Moreover, we found that depletion of MKL1 alone resulted in a marked increase in the expression of PPARγ and PPARγ target genes even in NIH 3T3 nonadipogenic fibroblasts ( Fig. 4b ; Supplementary Fig. 5a ). These findings indicated that loss of MKL1 function elicits PPARγ expression and adipocyte differentiation in vitro . 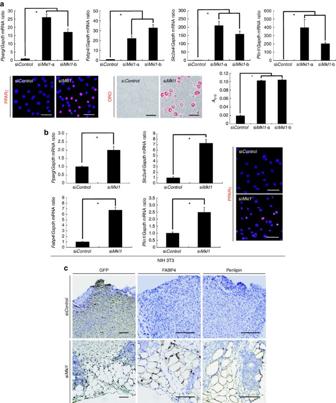Figure 4: Loss of MKL1 is sufficient to drive adipocyte differentiationin vitroandin vivo. (a) DFAT cells were transiently transfected with MKL1 (siMkl1-a or -b) or control (siControl) siRNAs for 48 h and then cultured in growth medium without an adipogenic cocktail for 96 h, after which the relative abundance ofPparg,Fabp4,Slc2a4andPlin1mRNAs was determined (upper panels). The cells were also subjected to immunofluorescence analysis of PPARγ expression (bottom left panel). Nuclei were stained with Hoechst 33342. Scale bars, 100 μm. They were also stained with oil red O (bottom centre panel; Scale bars, 100 μm), and theA510of dye extracted from the stained cells was determined (bottom right panel). (b) NIH 3T3 fibroblasts were transiently transfected with MKL1 (siMkl1-a) or control siRNAs for 48 h and then cultured in growth medium without an adipogenic cocktail for 96 h, after which the relative abundance ofPparg,Fabp4,Slc2a4, andPlin1mRNAs was determined (left panels). The cells were also subjected to immunofluorescence analysis of PPARγ expression (right panel). Nuclei were stained with Hoechst 33342. Scale bars, 100 μm. (c) DFAT cells were transiently transfected with MKL1 (siMkl1-a) or control siRNAs for 48 h and then injected subcutaneously into mice. Serial sections of the injection site were subjected to immunohistochemical staining of GFP (to identify injected cells) as well as of FABP4 and perilipin (markers of terminal adipogenic differentiation) at 2 weeks after injection. The sections were counterstained with hematoxylin. Data are representative of five mice per group. Scale bars, 100 μm. All quantitative data are means±s.d. (n=3 experiments). *P<0.05, Student’st-test. Figure 4: Loss of MKL1 is sufficient to drive adipocyte differentiation in vitro and in vivo . ( a ) DFAT cells were transiently transfected with MKL1 (si Mkl1 -a or -b) or control (si Control ) siRNAs for 48 h and then cultured in growth medium without an adipogenic cocktail for 96 h, after which the relative abundance of Pparg , Fabp4 , Slc2a4 and Plin1 mRNAs was determined (upper panels). The cells were also subjected to immunofluorescence analysis of PPARγ expression (bottom left panel). Nuclei were stained with Hoechst 33342. Scale bars, 100 μm. They were also stained with oil red O (bottom centre panel; Scale bars, 100 μm), and the A 510 of dye extracted from the stained cells was determined (bottom right panel). ( b ) NIH 3T3 fibroblasts were transiently transfected with MKL1 (si Mkl1 -a) or control siRNAs for 48 h and then cultured in growth medium without an adipogenic cocktail for 96 h, after which the relative abundance of Pparg , Fabp4 , Slc2a4 , and Plin1 mRNAs was determined (left panels). The cells were also subjected to immunofluorescence analysis of PPARγ expression (right panel). Nuclei were stained with Hoechst 33342. Scale bars, 100 μm. ( c ) DFAT cells were transiently transfected with MKL1 (si Mkl1 -a) or control siRNAs for 48 h and then injected subcutaneously into mice. Serial sections of the injection site were subjected to immunohistochemical staining of GFP (to identify injected cells) as well as of FABP4 and perilipin (markers of terminal adipogenic differentiation) at 2 weeks after injection. The sections were counterstained with hematoxylin. Data are representative of five mice per group. Scale bars, 100 μm. All quantitative data are means±s.d. ( n =3 experiments). * P <0.05, Student’s t -test. Full size image To investigate the function of MKL1 in adipocyte differentiation in vivo , we transfected DFAT cells (which are derived from green fluorescent protein (GFP) transgenic mice) [12] with MKL1 siRNA for 48 h (resulting in a significant decrease in Mkl1 expression but no change in Pparg expression at this time ( Supplementary Fig. 5d )) and then injected the cells subcutaneously into mice. At 2 weeks after injection, many fully differentiated adipocytes were observed at the injection site in the animals that received cells transfected with MKL1 siRNA but not in those that received cells transfected with a control siRNA ( Fig. 4c ). The transplanted MKL1-depleted cells were thus strongly positive for markers of terminal adipogenic differentiation (FABP4 and perilipin) as well as for GFP ( Fig. 4c ). Together, these data revealed that MKL1 functions as a gatekeeper that controls adipocyte differentiation both in vitro and in vivo . It was previously reported that the postpartum mammary glands of Mkl1 knockout female mouse show premature involution and markedly increased white adipose tissue [34] . This phenotype of Mkl1 knockout mouse is concordant with our finding that loss of Mkl1 promotes adipocyte differentiation programme. We also performed microarray analysis to examine the gene expression profile of cells treated with ROCK inhibitor (Y-27632) or depleted MKL1 expression by siRNA (siMkl1) and functional classification of highly expressed genes (>2-fold). The gene ontology (GO) analysis revealed the most significant biological function was ‘fat cell differentiation’ (GO:0045444) in both ROCK inhibition and MKL1 knockdown ( Table 1 ). Furthermore, hierarchical clustering of all samples for 133 fat cell differentiation-associated genes demonstrated an extremely high similarity of the gene expression pattern between Y-27632 sample and siMkl1 sample ( Supplementary Fig. 6a ), suggesting that either ROCK inhibition or MKL1 knockdown alone predominantly induces the expression of adipocyte differentiation-associated genes in global gene expression level. Furthermore, we extracted the expression patterns of a large number of well-documented serum response factor (SRF)-MKL1 target genes [26] from those microarray data. The relative expression of these SRF-MKL1 target genes tends to decrease on ROCK inhibition and MKL1 knockdown ( Supplementary Fig. 6b ), suggesting that either ROCK inhibition or MKL1 knockdown in common suppresses the expression of genes downstream of MKL1. Table 1 Gene ontology classifications for the highly expressed genes in ROCK inhibitor or MKL1 knockdown. Full size table PPARγ induces Mkl1 downregulation during adipogenesis We noticed that treatment with Y-27632, which elicited remodelling of the actin cytoskeleton, not only prevented nuclear translocation of MKL1 but also induced a significant decrease in the amount of Mkl1 mRNA in DFAT cells and 3T3-L1 preadipocytes ( Supplementary Fig. 3i ). Moreover, we found that Mkl1 expression correlated inversely with Pparg expression during adipocytic differentiation ( Fig. 5a ). To test whether PPARγ contributes to Mkl1 downregulation during adipogenesis, we investigated the effect of PPARγ knockdown on Mkl1 expression. We established DFAT cells stably depleted of PPARγ as a result of retrovirus-mediated expression of a specific short hairpin RNA (shRNA) ( Fig. 5b ). Although control cells expressing a luciferase shRNA manifested a significant decrease in the abundance of Mkl1 mRNA after exposure to inducers of adipocytic differentiation, cells expressing the PPARγ shRNA did not ( Fig. 5b ). To clarify further the influence of PPARγ on Mkl1 expression, we generated DFAT cells that stably overexpress PPARγ ( Fig. 5c ). Overexpression of PPARγ resulted in a significant decrease in the amount of Mkl1 mRNA ( Fig. 5c ), indicating that PPARγ indeed suppresses the expression of Mkl1 , resulting in the continuous activation of PPARγ required for the completion of adipocyte differentiation. 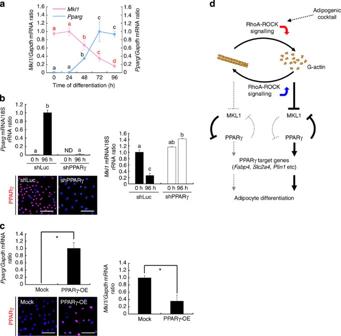Figure 5: PPARγ contributes toMkl1downregulation during adipocyte differentiation. (a) The relative abundance ofMkl1andPpargmRNAs at the indicated times after exposure of DFAT cells to inducers of adipocytic differentiation was also determined. (a–c)P<0.05, (a–d)P<0.05, Tukey’s honest significant difference test. (b) DFAT cells stably expressing PPARγ (shPPARγ) or luciferase (shLuc, control) shRNAs were exposed to inducers of adipogenesis for 0 or 96 h and then assayed for the relative abundance ofPpargandMkl1mRNAs. The cells were also subjected to immunofluorescence analysis of PPARγ after 96 h. Nuclei were stained with Hoechst 33342. Scale bars, 100 μm. ND, not detected. (c) DFAT cells stably overexpressing PPARγ (PPARγ-OE) or infected with the corresponding empty vector (Mock) were assayed for the relative abundance ofPpargandMkl1mRNAs. *P<0.05, Student’st-test. They were also subjected to immunofluorescence analysis of PPARγ expression. Nuclei were stained with Hoechst 33342. Scale bars, 100 μm. All quantitative data are means±s.d. (n=3 experiments). (d) Model for the regulation of adipocyte differentiation. Regulation of MKL1 by disruption of actin stress fibres drives adipocyte differentiation. Figure 5: PPARγ contributes to Mkl1 downregulation during adipocyte differentiation. ( a ) The relative abundance of Mkl1 and Pparg mRNAs at the indicated times after exposure of DFAT cells to inducers of adipocytic differentiation was also determined. ( a – c ) P <0.05, ( a – d ) P <0.05, Tukey’s honest significant difference test. ( b ) DFAT cells stably expressing PPARγ (shPPARγ) or luciferase (shLuc, control) shRNAs were exposed to inducers of adipogenesis for 0 or 96 h and then assayed for the relative abundance of Pparg and Mkl1 mRNAs. The cells were also subjected to immunofluorescence analysis of PPARγ after 96 h. Nuclei were stained with Hoechst 33342. Scale bars, 100 μm. ND, not detected. ( c ) DFAT cells stably overexpressing PPARγ (PPARγ-OE) or infected with the corresponding empty vector (Mock) were assayed for the relative abundance of Pparg and Mkl1 mRNAs. * P <0.05, Student’s t -test. They were also subjected to immunofluorescence analysis of PPARγ expression. Nuclei were stained with Hoechst 33342. Scale bars, 100 μm. All quantitative data are means±s.d. ( n =3 experiments). ( d ) Model for the regulation of adipocyte differentiation. Regulation of MKL1 by disruption of actin stress fibres drives adipocyte differentiation. Full size image On the basis of our observations, we propose a model for the control of adipocyte differentiation in which regulation of MKL1 by disruption of actin stress fibres triggers the differentiation programme ( Fig. 5d ). Exposure of preadipocytes to an adipogenic cocktail results in the rapid disruption of actin stress fibres as a consequence of downregulation of RhoA-ROCK signalling. The resulting increase in the amount of G-actin leads to the binding of G-actin to MKL1 and to inhibition of the nuclear translocation and transcriptional regulatory activity of the latter protein. Transcription of the Pparg gene is thereby activated, and the encoded protein then mediates not only upregulation of the expression of genes (such as Fabp4 , Plin and Slc2a4 ) associated with the adipocyte phenotype but also downregulation of Mkl1 expression to allow completion of adipogenesis. Several preadipocyte cell lines undergo differentiation on treatment with a standard adipogenic cocktail consisting of IBMX, dexamethasone and insulin [35] . Both IBMX and dexamethasone trigger the activation of protein kinase A by increasing the intracellular concentration of cAMP, thereby promoting adipocyte differentiation [36] . The major role of protein kinase A in adipogenesis has been thought to lie in downregulation of RhoA and ROCK activity [37] . In the present study, we found that Rho activity is rapidly reduced after treatment of DFAT cells with the adipogenic cocktail, and the downregulation of RhoA-ROCK signalling then promotes adipocyte differentiation via modulation of remodelling of the actin cytoskeleton. In addition, we found that treatment with LatA alone or Y-27632 alone, by inducing remodelling of the actin cytoskeleton, is sufficient to trigger adipocyte differentiation in the absence of an adipogenic cocktail. Our findings, combined with previous observations, thus suggest that a standard adipogenic cocktail directly elicits reorganization of the actin cytoskeleton through downregulation of RhoA-ROCK signalling, and that the disruption of actin stress fibres then acts as a trigger for the adipocytic differentiation of preadipocytes in vitro . In differentiated adipocytes, cortical F-actin has an important regulatory role in the insulin-stimulated translocation of the glucose transporter GLUT4 (encoded by Slc2a4 ) from intracellular storage sites to the plasma membrane [10] , with the formation of cortical F-actin thus likely being a key event in adipogenesis. In the present study, F-actin stress fibres were depolymerized to G-actin within 24 h after the induction of adipocyte differentiation, and the actin cytoskeleton was subsequently reorganized to form cortical F-actin structures within 48 h. The abundance of transcripts for MKL1, which binds to G-actin, began to decline within 48 h after induction of adipocyte differentiation, and this downregulation of Mkl1 was controlled by PPARγ. We also found that cells depleted of PPARγ maintained a high level of Mkl1 expression even after induction of adipocyte differentiation, and that these cells manifested disruption of actin stress fibres at 24 h but not the formation of cortical F-actin structures even at 96 h ( Supplementary Fig. 4e ). Together, these observations suggest that the downregulation of Mkl1 expression not only contributes to the continued activation of PPARγ but also promotes the organization of adipocyte-specific cortical F-actin structures as a result of the release of G-actin from MKL1–G-actin complexes. Our findings provide new insight into the regulatory mechanism of adipocyte differentiation, which is shown to be triggered through regulation of MKL1 resulting from disruption of actin stress fibres. They also identify MKL1 as a novel gatekeeper in the regulation of adipogenesis as well as provide a basis for further studies of the relation between the dynamics of cell shape and transcription factor function during cellular differentiation. Lastly, given that activating mutations of RAC protein, which belongs to the RHO family of small GTPases and orchestrates actin polymerization, were found in a wide variety of human cancers and given their marked transforming ability [38] , we assume that aberrant differentiation associated with actin cytoskeleton dynamics can be a critical factor of tumorigenesis, and our works thus would potentially contribute to understanding cancer biology. Cell culture The mouse preadipocyte cell line DFAT was established from dedifferentiated mature adipocytes of GFP transgenic mice by ceiling culture (a method to culture lipid-containing adipocytes based on their lipid buoyancy) [12] . The mouse embryonic preadipocyte cell line 3T3-L1 and the mouse embryonic fibroblast cell line NIH 3T3 were obtained from the Japanese Collection of Research Bioresources (Tokyo, Japan). DFAT, 3T3-L1, or NIH 3T3 cells were cultured under a humidified atmosphere of 5% CO 2 and 95% air at 37 °C on glass coverslips (Matsunami, Osaka, Japan) placed in tissue culture dishes (Falcon 3001; BD, Bedford, MA) containing Dulbecco’s modified Eagle’s medium (DMEM) (Nissui Pharmaceutical, Tokyo, Japan) supplemented with 10% fetal bovine serum (FBS) (Moregate BioTech, Bulimba, Queensland, Australia). DFAT or 3T3-L1 cells were grown to semiconfluence before induction of differentiation by exposure to DMEM supplemented with FBS (1% or 10%, respectively), 0.5 mM IBMX (Wako, Osaka, Japan), 0.1 μM dexamethasone (Wako), and insulin-transferrin-selenium-X supplement (final insulin concentration of 5 μg ml −1 ) (Invitrogen, Carlsbad, CA). Time-lapse imaging For time-lapse observation of actin dynamics during adipocyte differentiation, DFAT cells were infected with Cellular Lights Actin-RFP baculovirus expression vectors (Invitrogen) and then cultured in a glass-bottomed dish (Iwaki, Chiba, Japan). After the cells achieved semiconfluence, adipocyte differentiation was induced as described above and time-lapse fluorescence and differential interference contrast video microscopy was performed with the use of a microscope (Olympus LCV110) equipped with an incubation chamber. Images were acquired every 30 min with the use of a charge-coupled device camera (Retiga Exi, QImaging) equipped with a U Plan Super Apochromatic × 40, 0.95 numerical aperture objective and were analysed with MetaMorph software (Molecular Devices, Sunnyvale, CA). RT and real-time PCR analysis Total RNA was isolated from cells with the use of the Trizol reagent (Invitrogen), and portions (1 μg) of the DNase I–treated RNA were subjected to reverse transcription (RT) with the use of high-capacity RNA-to-cDNA master mix (Applied Biosystems, Foster City, CA). The probes for PPARγ ( Pparg ; GenBank accession no. NM_011146.3; Mm00440940_m1), C/EBPα ( Cebpa ; GenBank accession no. NM_007678.3; Mm00514283_s1), fatty acid-binding protein 4 ( Fabp4 ; GenBank accession no. NM_024406.2; Mm00445878_m1), GLUT4 ( Slc2a4 ; GenBank accession no. NM_009204.2; Mm01245502_m1), perilipin 1 ( Plin1 ; GenBank accession no. NM_175640.2; Mm00558672_m1) and MKL1 ( Mkl1 ; GenBank accession no. NM_153049.2; Mm00461840_m1) genes were obtained fromTaqMan Pre-Developed Assay Reagents (Applied Biosystems). A mouse glyceraldehyde-3-phosphate dehydrogenase ( Gapdh ; GenBank accession no. NM_008084.2) TaqMan probe (4352339E, Applied Biosystems) or eukaryotic 18S rRNA (GenBank accession no. X03205.1) TaqMan probe (4319413E, Applied Biosystems) was included as an endogenous control. The RT products (2 μl) were subjected to real-time PCR analysis in a final volume of 10 μl with the use of TaqMan Fast Universal PCR master mix (Applied Biosystems) and with an ABI7500 thermocycler. Each sample was assayed in triplicate. Immunoblot analysis Cells were washed extensively with phosphate-buffered saline (PBS) and then either recovered directly with a rubber scraper in SDS sample buffer (62.5 mM Tris-HCl (pH 6.8), 10% SDS, 5% glycerol, 5% β-mercaptoethanol, 10% bromophenol blue) or subjected to extraction of nuclear and cytoplasmic fractions with the use of an NE-PER nuclear and cytoplasmic extraction reagent kit (Pierce, Rockford, IL). Samples were subjected to SDS–polyacrylamide gel electrophoresis, the separated proteins were transferred electrophoretically to a polyvinylidene difluoride membrane (Millipore, Bedford, MA), and nonspecific sites of the membrane were then blocked by incubation with Blocking One (Nacalai Tesque, Kyoto, Japan) for 1 h at room temperature. The membrane was then exposed for 24 h at 4 °C to rabbit polyclonal antibodies to PPARγ (1:500 dilution; P0744; Sigma-Aldrich, St Louis, MO), to lamin A/C (1:500 dilution; #2032; Cell Signalling Technology, Beverly, MA), or to MEK1/2 (1:500 dilution; #9122; Cell Signalling Technology); rabbit monoclonal antibodies to cofilin (1:1,000 dilution; #5175; Cell Signalling Technology); or mouse monoclonal antibodies to FLAG (1:1,000 dilution; F1804; Sigma-Aldrich), to GAPDH (1:10,000 dilution; G8795; Sigma-Aldrich), or to α-tubulin (1:10,000 dilution; T5168; Sigma-Aldrich). The membrane was washed with PBS containing 0.02% Tween 20, incubated for 1 h at room temperature with horseradish peroxidase–conjugated goat antibodies to rabbit or mouse immunoglobulin G (1:2,000 dilution; GE Healthcare, Tokyo, Japan), and washed again with PBS containing 0.02% Tween 20, after which immunoreactive proteins were visualized with the use of enhanced chemiluminescence reagents (GE Healthcare). Uncropped scans of the most important western blots were shown in Supplementary Fig. 7 . Immunofluorescence staining Cells were fixed overnight at 4 °C in zinc fixative solution (0.1 M Tris-HCl (pH 7.4), calcium acetate (475 μg ml −1 ), zinc acetate (5 mg ml −1 ) and ZnCl 2 (5 mg ml −1 ) in ultrapure water) containing 0.2% Triton X-100. They were then washed in Tris-buffered saline (TBS) and incubated for 1 h at room temperature with 10% normal goat or horse serum (Vector Laboratories, Burlingame, CA) and 1% bovine serum albumin (BSA) (Sigma-Aldrich) in TBS to block nonspecific binding of antibodies before staining with primary antibodies according to standard procedures. Primary antibodies included rabbit monoclonal antibodies to PPARγ (1:200 dilution; #2435; Cell Signalling Technology); rabbit polyclonal antibodies to perilipin A/B (1:1,000 dilution; P1873; Sigma-Aldrich) and to MKL1 (1:100 dilution; ab49311; Abcam, Cambridge, MA); and mouse monoclonal antibodies to β-actin (1:1,000 dilution; A5441; Sigma-Aldrich), to HA (1:500 dilution; 1583816; Roche, Mannheim, Germany), and to FLAG (1:1,000 dilution; F1804; Sigma-Aldrich). Immune complexes were detected with Alexa Fluor 488– or Alexa Fluor 594–conjugated goat antibodies to rabbit or mouse immunoglobulin G (each at 1:2,000 dilution; Molecular Probes, Eugene, OR). Antibodies were diluted in TBS containing 1% BSA. F-actin was stained with Alexa Fluor 488– or Alex Fluor 594–labelled phalloidin (Molecular Probes) at 200 U ml −1 in TBS, and G-actin was stained with Alexa Fluor 594–labelled DNase I (Molecular Probes) at 9 μg ml −1 in TBS. Cells were counterstained with Hoechst 33342 (Sigma-Aldrich) at 5 μg ml −1 in TBS and were observed with a laser-scanning confocal microscope (Olympus FV-750) and a BIOREVO BZ-9000 fluorescence microscope (Keyence, Osaka, Japan). Lipid staining Lipid accumulation in adipocytes was detected by staining with oil red O (Wako). Cells were washed three times with PBS, fixed for 1 h at room temperature with 10% formalin in phosphate buffer, washed again with PBS and stained for 15 min at room temperature with a filtered solution of oil red O (0.5 g in 100 ml of isopropyl alcohol). The cells were then washed twice with distilled water for 15 min. For quantitation of lipid accumulation, dimethyl sulfoxide (DMSO) (500 μl per 35-mm dish) was added to the washed and dried cells for 1 min, after which the absorbance of the extracted dye at 510 nm was measured with a spectrophotometer (ND-1000; Nanodrop Technologies, Wilmington, DE) and was normalized by dish area. Pharmacological agents Cells were exposed to the following agents: 5 μM phalloidin oleate (Calbiochem, San Diego, CA) dissolved in DMSO, 30 μM Y-27632 (Calbiochem) dissolved in water, 0.2 μM cytochalasin D (CytD) (Sigma-Aldrich) dissolved in DMSO, 0.4 μM latrunculin A (LatA) (Calbiochem) dissolved in DMSO, 0.1 μM swinholide A (SwinA) (Calbiochem) dissolved in ethanol or 1 μM 4-hydroxytamoxifen (TAM) (Sigma-Aldrich) dissolved in ethanol. Rho activation assay Cells were lysed by incubation with a magnesium-containing buffer (25 mM HEPES-NaOH (pH 7.5), 150 mM NaCl, 1% Igepal CA-630 detergent, 10 mM MgCl 2 , 1 mM EDTA, 2% glycerol) supplemented with 25 mM NaF, 1 mM Na 3 VO 4 , and a protease inhibitor cocktail (Nacalai Tesque). The lysates were centrifuged at 14,000 × g for 5 min at 4 °C, and the resulting supernatants were incubated for 45 min at 4 °C with 25 μg of a glutathione S-transferase fusion protein of the Rho-binding domain (amino acids 7–89) of rhotekin that was bound to glutathione-Sepharose beads (Millipore). The beads were washed three times with the magnesium-containing buffer and then subjected to immunoblot analysis with mouse monoclonal antibodies to RhoA, -B and -C (1:250 dilution; #05-778; Millipore). Whole-cell lysates were also subjected to immunoblot analysis with the antibodies to Rho and those to GAPDH (loading control). Transplantation and histological evaluation All animal studies were performed according to the NIH Guide for the Care and Use of Laboratory Animals. C57BL/6J mice were obtained from Oriental Yeast (Tokyo, Japan). DFAT cells (1 × 10 5 ) collected with the use of a cell scraper were injected subcutaneously with a syringe above the sternum of 10 female mice at 8 weeks of age. After 2 weeks, cells at the injection site were retrieved, fixed in paraformaldehyde and embedded in paraffin. For immunohistochemical analysis, tissue sections were depleted of paraffin, washed with TBS, and stained with the use of a Vectastain ABC kit (Vector Laboratories). Primary antibodies included rabbit polyclonal antibodies to GFP (1:100 dilution; sc-8334; Santa Cruz Biotechnology, Santa Cruz, CA), to FABP4 (1:1,000 dilution; ab13979; Abcam) and to perilipin A/B (1:1,000 dilution; P1873; Sigma-Aldrich). The sections were counterstained with hematoxylin (Wako). Plasmid transfection The plasmids pEF-BOS-HA-RhoAV14 and pEF-BOS-HA-RhoAN19 (ref. 39 ) plasmids were transfected into DFAT cells for 24 h using the Fugene HD reagent (Roche). RNAi Expression of shRNAs was achieved with the retroviral expression vector pRePS (kindly provided by T. Hara), which also contains a puromycin resistance gene. The sequences of the sense oligonucleotides were 5′-GTTTGAGTTTGCTGTGAAG-3′ for PPARγ shRNA [40] and 5′-CGTACGCGGAATACTTCGA-3′ for luciferase shRNA (nonspecific control). pReps vectors transfected into Plat-E packaging cells [41] using Fugene HD (Roche). Medium was replaced once after 24 h, and viral supernatants were collected and filtered with 0.45-μm cellulose acetate filters (Iwaki) 48 h after transfection. Retroviral infection was carried out in a six-well plate for 48 h, and infected cells were then subjected to selection in the presence of puromycin (10 μg ml −1 ). The sequences of siRNAs targeting cofilin1 were 5′-GAUGAACACCAGGUCCUCCUU-3′ for Cfl1 -a, 5′-AAGAUCAAAAGCAGUUUGGGA-3′ for Cfl1 -b, and 5′-UCACUAUUGUGGUUAGAAGUU-3′ for Cfl1 -c, and those of siRNAs targeting MKL1 were 5′-CGAGGACUAUUUGAAACGGAA-3′ for Mkl1 -a and 5′-CCCACUCAGGUUCUUUCUCAA-3′ for Mkl1 -b. The control siRNA sequence was 5′-GCGCGCUUUGUAGGAUUCG-3′. Cells were transfected with siRNA duplexes for 48 h with the use of Lipofectamine RNAiMAX (Invitrogen). Retroviral gene transfer The coding region for mCherry cDNA was amplified from the vector containing mCherry-MKlp2 (ref. 42 ) by PCR with the primers 5′-CCGCTCGAGATGGTGAGCAAGGGCGAGGAGGATAACATG-3′ (XhoI_mCherry forward primer) and 5′-CGGAATTCTTCTTGTACAGCTCGTCCATGCCGCCGGTGG-3′ (mCherry_EcoRI reverse primer), and the coding region for human ER was amplified from the pMV7-MycER plasmid [43] by PCR with the primers 5′-CCGCTCGAGTCTGCTGGAGACATGAGAGCTGCCAACCTT-3′ (XhoI_ER forward primer) and 5′-CGGAATTCTTGACCGTGGCAGGGAAACCCTCTGCCTCCCC-3′ (ER_EcoRI reverse primer), digested with XhoI and EcoRI, and ligated into the XhoI and EcoRI sites of pMXs-3 × FLAG-IP [42] . Human cDNAs for full-length MKL1 and MKL1-N100 were obtained by digestion of Addgene Plasmids (#11978, #27176) [32] with EcoRI and BamHI, and the resulting fragments were cloned into the EcoRI and BamHI sites of pMXs-3 × FLAG-mCherry-IP and/or pMXs-3 × FLAG-ER-IP. The resulting vectors were designated pMXs-3 × FLAG-mCherry-MKL1-IP, pMXs-3 × FLAG-ER-MKL1-IP, or pMXs-3 × FLAG-ER-MKL1-N100-IP, and pMXs-3 × FLAG-mCherry-IP or pMXs-3 × FLAG-ER-IP was used as a control. Mouse PPARγ cDNA (ImaGenes, Berlin, Germany) was cloned into the retroviral plasmid pMXs-puro (kindly provided by T. Kitamura). pMXs vectors were transfected into Plat-E packaging cells [44] using FugeneHD (Roche). Medium was replaced once after 24 h, and viral supernatants were collected and filtered with 0.45-μm cellulose acetate filters (Iwaki) 48 h after transfection. Retroviral infection was carried out in a six-well plate for 48 h, and infected cells were subjected to selection in the presence of puromycin (10 μg ml −1 ). Microarray analysis The quality of RNA was assessed using the Agilent 2100 Bioanalyzer (Agilent Technologies, Waldbronn, Germany). The RNA samples were labelled using the GeneChip One-Cycle Target Labeling and Control Reagent pakage (Affymetrix, Santa Clara, CA) and then hybridized to the Affymetrix GeneChip mouse genome 430 2.0 array according to the manufacturer’s instruction. Fluorescent images were visualized using a GeneChip Scanner 3000 (Affymetrix). Expression and raw expression data (CEL files) were summarized and normalized using the Robust Multi-array Average algorithm and the Bioconductor package affy ( http://www.bioconductor.org/packages/2.0/bioc/html/affy.html ). The Spotfire DecisionSite for Functional Genomics software package (TIBCO Software, Palo Alto, CA) was used for visualization of microarray data. Functional analyses were performed using DAVID Bioinformatics Resources 6.7 ( http://david.abcc.ncifcrf.gov/ ). Functional analysis identified the biological functions that were most significant to the data set. Statistical analysis Data are presented as means±s.d. and were analysed with Tukey’s honest significant difference test or Student’s t -test for comparisons between two or among three or more groups, respectively. A P -value of <0.05 was considered statistically significant. How to cite this article: Nobusue, H. et al. Regulation of MKL1 via actin cytoskeleton dynamics drives adipocyte differentiation. Nat. Commun. 5:3368 doi: 10.1038/ncomms4368 (2014). Accession codes: The raw and processed microarray data have been deposited in the Gene Expression Omnibus under the accession code GSE52334 .